Characterizing the interplay between multiple levels of organization within bacterial sigma factor regulatory networks Bacteria contain multiple sigma factors, each targeting diverse, but often overlapping sets of promoters, thereby forming a complex network. The layout and deployment of such a sigma factor network directly impacts global transcriptional regulation and ultimately dictates the phenotype. Here we integrate multi-omic data sets to determine the topology, the operational, and functional states of the sigma factor network in Geobacter sulfurreducens , revealing a unique network topology of interacting sigma factors. Analysis of the operational state of the sigma factor network shows a highly modular structure with σ N being the major regulator of energy metabolism. Surprisingly, the functional state of the network during the two most divergent growth conditions is nearly static, with sigma factor binding profiles almost invariant to environmental stimuli. This first comprehensive elucidation of the interplay between different levels of the sigma factor network organization is fundamental to characterize transcriptional regulatory mechanisms in bacteria. The core RNA polymerase in bacteria consists of five core subunits (α2ββ′ω) and a dissociable sixth subunit, the sigma factor (σ), which is critical for transcriptional initiation. When a given σ factor associates with the core RNA polymerase, the resulting holoenzyme acquires the ability to recognize promoter motifs and initiate transcription. Bacteria typically contain a housekeeping σ factor that is responsible for initiation of transcription from the majority of promoters. Additionally, bacteria encode several to dozens of alternative σ factors that control transcriptional initiation of a subset of genes [1] . The number and utilization of these alternative σ factors varies widely among different bacterial species, and is related to the diversity of lifestyles [1] , [2] . For example, while Escherichia coli, encodes 7 σ factors, the soil bacterium Streptomyces coelicolor contains 60 alternative σ factors [1] . These different σ factors often interact with each other by targeting overlapping sets of promoters, thereby resulting in a complex regulatory network to modulate the variety of cellular processes [3] . Several approaches, mostly computational, have been employed to determine binding sites to elucidate the regulatory network [4] , [5] , [6] . These computational methods, however, do not account for condition-specific binding information, and thus cannot determine the functional state of the network. Therefore, experimental methods, such as chromatin immunoprecipitation coupled to microarray (ChIP-chip) or to sequencing (ChIP-seq), have recently been applied to determine condition-specific binding of σ factors to DNA directly [7] , [8] . Recently, we demonstrated the utility of a systems approach that integrates a diversity of multi-omic data sets to characterize the structural, operational, and functional organizations of the genomes of the generalist E. coli and the specialist Geobacter sulfurreducens [9] , [10] . Here, we elucidated the comprehensive σ factor network in G. sulfurreducens , a bacterium that has been studied extensively for its impact on the natural environment and its capability of electricity production from organic waste [11] , [12] . The network of the four major σ factors in G. sulfurreducens (σ D , σ H , σ N and σ S ) was resolved by combining experimentally determined σ factor binding with computational approaches in the context of the previously described transcriptional unit architecture [9] . In addition to determining the topology of the G. sulfurreducens σ factor network, we characterized its operational state and its effect on the physiological functional state of the cell. This comprehensive multi-level characterization of σ factor regulons and their complex regulatory network serves as the scaffold necessary to build the entire transcriptional regulatory network. σ factor network topology in G. sulfurreducens G. sulfurreducens encodes six different σ factors. In addition to the housekeeping σ D (RpoD), it also contains the extracytoplasmic stress σ E (RpoE), the flagellar σ F (RpoF), the heat stress σ H (RpoH), the nitrogen limitation related σ N (RpoN) and the stress- and starvation-induced σ S (RpoS). The network topology of the σ factor network was determined using a ChIP-chip approach to obtain genome-wide binding profiles for the four major σ factors σ D , σ H , σ N and σ S under various growth conditions ( Supplementary Data 1 ). Binding profiles of σ D , σ N and σ S were obtained from cells grown with acetate as electron donor either planktonically with fumarate or as a biofilm on an electrode serving as the terminal electron acceptor. Furthermore, σ factor binding profiles were obtained under the specific conditions, where their activity has been previously documented [13] , [14] . Specifically, binding profiles of σ H and σ N were obtained from cells under heat shock stress and nitrogen limitation, respectively. σ F was excluded from this study as the 32 flagella genes controlled by this σ factor were found to be usually silent [15] , [16] . Although several conditions were assayed for σ E , no suitable condition could be obtained to induce its expression. Binding peaks for σ D , σ H , σ N and σ S under various conditions were identified by applying peak-calling algorithms (NimbleScan and MA2C [17] ) to ChIP-chip data sets. Peaks that were identified by both algorithms with at least two-fold enrichment were considered binding regions (see Methods). These bona fide binding regions were subsequently mapped to the previously elucidated transcription unit architecture of G. sulfurreducens [9] to determine the regulon of each σ factor. 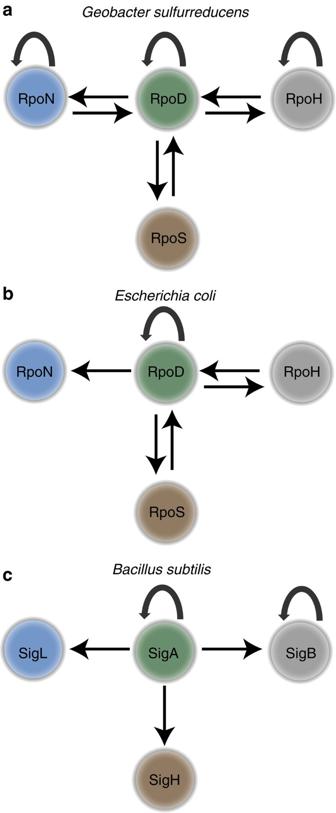Figure 1: σ factor network topology. (a) The topology of the interaction network of the four major σ factors inG. sulfurreducens.(b) The topology of the interaction network of the four major σ factors inE. coli(based on RegulonDB44). (c) The topology of the interaction network of the four major σ factors inB. subtilis(based on BsubCyc and Nicolaset al.18,19). InB. subtilis, SigA is equivalent to RpoD, SigB to RpoH, SigL to RpoN and SigH to RpoS18. Overall, a total of 1,522 binding regions were identified in the G. sulfurreducens genome ( Table 1 ; Supplementary Data 1 ). These binding regions were mapped onto the promoter regions of 1,339 transcription units, covering >80% (2,620 genes) of all genes. A total of 652 binding regions were identified for σ D , which controlled transcription of ~60% of the genome (2,050 genes), confirming the role of σ D as housekeeping σ factor. Table 1 Regulons of σ factors in Geobacter sulfurreducens . Full size table Multiple genome-wide binding sites for σ H (275), σ N (349) and σ S (246) were identified. These binding sites controlled transcription of 802 (σ H ), 909 (σ N ) and 863 (σ S ) genes ( Table 1 ). We confirmed many genes previously described to be regulated by σ H , such as heat-inducible chaperones (for example, hspA ) [13] , or by σ N , such as the nitrogenase molybdenum-iron cofactor biosynthesis protein ( nifEN ) [14] . In addition to nifEN being transcribed from a σ N -specific promoter, σ N was the only σ factor controlling this essential gene for nitrogen fixation. These results are consistent with previously identified regulons of these σ factors [1] . Each alternative σ factor in G. sulfurreducens directly regulates ~25% of the ORFs ( Table 1 ), suggesting a broader role for these alternative σ factors in G. sulfurreducens . The topology of the G. sulfurreducens σ factor network indicated a robust network with all alternative σ factors (σ H , σ N and σ S ) regulating the housekeeping σ D ( Fig. 1a ). Specifically, σ N is found to auto-regulate itself and regulate σ D , thereby suggesting a pronounced role for σ N in addition to σ D . In contrast, σ H , σ N and σ S in E. coli and Bacillus subtilis exhibit different topologies ( Fig. 1b ). Neither σ H nor σ N auto-regulate themselves in E. coli and σ N does not regulate σ D . The Gram-positive bacterium B. subtilis has numerous (16) alternative σ factors. Despite this increased complexity in the σ factor network ( Supplementary Fig. S1 ) [18] , [19] , no alternative σ factor in B. subtilis regulated the expression of SigA (σ D equivalent) except for the sporulation σ factors SigEF. Similar to E. coli , neither SigL (σ N equivalent) nor SigH (post-exponential phase σ factor, σ S equivalent) auto-regulate themselves in B. subtilis ( Fig. 1c ; Supplementary Fig. S1 ). Thus, the intertwined topology and the auto-regulatory aspect of the σ factor network enable G. sulfurreducens to tightly regulate the expression levels of σ factors through feedback mechanisms and thus impacting the operation of the network. Expression levels of these σ factors were found to be relatively stable across all growth conditions assayed ( Supplementary Table S1 ). This indicates that the change in promoter occupancy of σ factors is usually not modulated through the transcription levels of the σ factors, but by other mechanisms. For example, the expression changes of genes for nitrogen fixation under nitrogen limitation conditions are due to the expression of specific σ N dependent regulators [14] . However, the heat shock σ factor (σ H ) was highly induced upon temperature upshift, suggesting that regulation of gene expression upon heat shock resulted from higher expression of the rpoH gene. Figure 1: σ factor network topology. ( a ) The topology of the interaction network of the four major σ factors in G. sulfurreducens. ( b ) The topology of the interaction network of the four major σ factors in E. coli (based on RegulonDB [44] ). ( c ) The topology of the interaction network of the four major σ factors in B. subtilis (based on BsubCyc and Nicolas et al . [18] , [19] ). In B. subtilis , SigA is equivalent to RpoD, SigB to RpoH, SigL to RpoN and SigH to RpoS [18] . Full size image The operational state of the σ factor network To determine the operational state of the σ factor network, we performed a functional enrichment analysis for the regulons of all four major σ factors (σ D , σ H , σ N and σ S ). 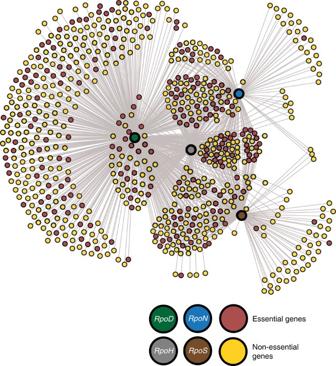Figure 2: Operational state of theG. sulfurreducensσ factor network. The interaction network of the four major σ factors with the metabolic genes inG. sulfurreducensis shown. Anin silicogene essentiality screen was carried out under four different conditions to assess the effect of genetic perturbations on the σ factor network operation. The genes determined to be essential under all four conditions are shown by red nodes; other non-essential genes are shown in gold. Genes with known functions were assigned to 24 subsystems based on the SEED database [20] , and a hypergeometric test was used to determine if a particular functional category is enriched in the regulon ( Table 2 ). The regulon of σ D was enriched in all major biosynthetic processes (nucleotide and amino-acid metabolism), and in cell wall and capsule synthesis. The regulon of the heat stress σ H was also enriched for nucleotide and amino-acid biosynthetic processes. The intertwined topology of the σ factor network was reflected in the enrichment for genes involved in membrane transport and protein metabolism in regulons of all four major σ factors. Expectedly, σ N was the main σ factor involved in regulating nitrogen metabolism. However, as hinted at by the topology of the network, the enrichment analysis revealed an expanded role for σ N in the operational state of the network. In addition to nitrogen metabolism, the σ N regulon was enriched for genes involved in other cellular processes, such as cell wall and capsule synthesis, and membrane transport. Most importantly, σ N was found to be the primary σ factor that regulates energy metabolism and respiration. Also, 18 genes that are transcribed from σ N -dependent promoters encode two component system genes, indicating its significant role in cell signalling and transcription regulation. These results suggest a much more pronounced role for σ N in G. sulfurreducens than previously described. σ S was the only other σ factor whose regulon was also enriched for genes involved in energy metabolism and respiration ( Table 2 ). This is likely because of its role in initiating the stationary growth phase, in which most energy-related processes are downregulated. Table 2 Enrichment of functional subsytems in G. sulfurreducens σ factor regulons. Full size table To assess the impact of the topology at the operational level, we investigated the effect of genetic perturbations on the operation of the σ factor network. As no validated essential gene list is available for G. sulfurreducens, we applied an in silico knock-out approach using a genome-scale metabolic model [21] , [22] . Such approaches have been successfully applied to predict gene essentiality [22] , [23] . A total of 809 genes present in the G. sulfurreducens metabolic reconstruction were individually knocked-out in silico , and growth simulations representing four different conditions were performed. These conditions included planktonic growth with either Fe(III) or fumarate as electron acceptor, growth as an electrogenic biofilm on an electrode, and planktonic growth under nitrogen limitation. A gene was considered essential if the corresponding in silico knock-out resulted in growth-deficient simulations in all four growth conditions. Most of the essential metabolic genes were under the control of σ D ( Fig. 2 ). Among the 229 essential genes identified, 75 of them were controlled solely by σ D , whereas over half of them (123) were regulated by σ D and at least one other alternative σ factor ( Supplementary Data 2 ). Only a handful of essential genes were not transcribed from a σ D promoter, but from an alternative σ factor promoter. For example, the gene GSU1745 that encodes the essential outer membrane porin OmpA [24] was only associated with a σ N -dependent promoter. This observation is consistent with the previously failed attempts to generate viable rpoN (σ N ) knock-out strains for G. sulfurreducens under multiple growth conditions [14] . Figure 2: Operational state of the G. sulfurreducens σ factor network. The interaction network of the four major σ factors with the metabolic genes in G. sulfurreducens is shown. An in silico gene essentiality screen was carried out under four different conditions to assess the effect of genetic perturbations on the σ factor network operation. The genes determined to be essential under all four conditions are shown by red nodes; other non-essential genes are shown in gold. Full size image In addition to the genes essential across all four conditions, several genes were determined to be essential only under certain specific conditions. Moreover, some of these genes were regulated solely by the housekeeping σ D and few of them were regulated by one of the alternative σ factors. For example, 7 out of 17 genes that are involved in nitrogen metabolism had only σ N -dependent promoters associated, and were found to be essential only under nitrogen limiting growth. These results highlight that although most cellular processes essential under all conditions are regulated by σ D , certain condition-specific essential processes are controlled by alternative σ factors. Furthermore, 15 of the 229 essential genes had promoters associated with all four σ factors. These included genes encoding for ATP synthase, as well as genes involved in amino-acid and nucleoside biosynthesis. By utilizing multiple σ factors for the most critical genes in the metabolic pathways, cells are able to fine-tune expression levels under various conditions to easily adapt to environmental changes. A similar utilization of multiple σ factors was also observed for genes related to other crucial cellular processes that are not part of the metabolic reconstruction, including genes involved in transcriptional machinery, such as infA , infB (transcription initiation factors), nusA (transcription elongation factor), rho (transcription termination factor) and rpoD (σ D ) itself. This broader role for alternative σ factors in the operation of G. sulfurreducens ’ σ factor network is a likely reflection of its topology. In contrast to this feature of shared regulation of essential genes by alternative σ factors, most of the essential genes in E. coli were regulated by a single σ factor ( Supplementary Fig. S2 ). Functional effect of the σ factor network operation One of the important features of bacterial σ factor usage is the selective preference for use of different σ factors depending on the growth condition. For example, it is known in E. coli that the intracellular level of σ S is extremely low during exponential growth. Only when cells are in stationary phase, σ S accumulates in the cell, binds to promoters of its regulon and activates their expression [25] . To investigate the functional state of the σ factor network in G. sulfurreducens , we compared binding profiles of σ D , σ N and σ S and transcriptomic changes under different growth conditions. The largest change in the transcriptome among all conditions examined was observed between cells grown planktonically and as an electrogenic biofilm on an electrode. These two divergent physiological states resulted in a difference of expression (>2-fold, FDR <0.05) of ~10% of the genome (367 genes) between these conditions ( Fig. 3a ). 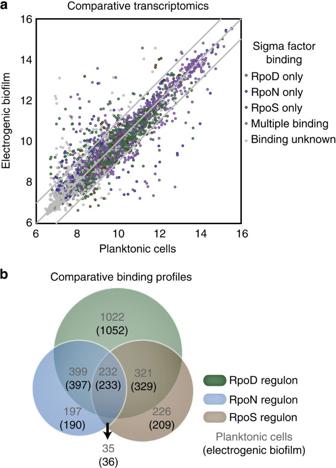Figure 3: Functional state of theG. sulfurreducensσ factor network. (a) Comparative transcriptomic profile betweenG. sulfurreducensgrown as planktonic cells reducing fumarate and as an electrogenic biofilm on an anode. About 10% of the transcriptome showed differential expression between the two conditions. Genes are highlighted based on binding profiles of σ factors in their promoters. (b) Venn diagram showing the comparative binding profiles of the three σ factors σD, σNand σSfor planktonic cells and electrogenic biofilm. The size of each σ factor regulon from electrogenic biofilm cells is shown in parentheses. The invariant binding profiles between the two conditions indicate a near-static functional state for the σ factor network inG. sulfurreducens. Expression levels of the σ factors were similar between different conditions (Supplementary Data 3). Figure 3: Functional state of the G. sulfurreducens σ factor network. ( a ) Comparative transcriptomic profile between G. sulfurreducens grown as planktonic cells reducing fumarate and as an electrogenic biofilm on an anode. About 10% of the transcriptome showed differential expression between the two conditions. Genes are highlighted based on binding profiles of σ factors in their promoters. ( b ) Venn diagram showing the comparative binding profiles of the three σ factors σ D , σ N and σ S for planktonic cells and electrogenic biofilm. The size of each σ factor regulon from electrogenic biofilm cells is shown in parentheses. The invariant binding profiles between the two conditions indicate a near-static functional state for the σ factor network in G. sulfurreducens . Expression levels of the σ factors were similar between different conditions ( Supplementary Data 3 ). Full size image Despite this change at the transcriptomic level, the overall binding profiles of the three σ factors during the shift between these two physiological states were surprisingly similar ( Fig. 3b ; Supplementary Fig. S3 ; Supplementary Data 1 and 3 ). All three σ factors were active in planktonic cells as well as in the biofilm. Genes under σ D control expanded from 1,974 genes in planktonic cells to 2,011 genes in electrogenic biofilm-forming cells. Compared with planktonic cells, 47 genes were under condition-specific regulation by σ D in the electrogenic biofilm. Utilization of the σ N regulon changed from 863 genes in planktonic cells to 856 under electrogenic biofilm growth, with 28 and 15 genes having condition-specifc σ N regulation, respectively. The number of genes under σ S control in exponentially grown planktonic cells (814 genes) was similar to the one for cells forming an electrogenic biofilm (807 genes), with two and 32 genes having condition-specific σ S regulation in electrogenic biofilm and planktonic cells, respectively. Next, we examined if these condition-specific bindings resulted in gene expression changes (>2-fold change, FDR <0.05). Under electronic biofilm growth, eight genes (five operons) have elevated transcription levels compared with planktonic cells and have electrogenic biofilm condition-specific σ factor bindings in their promoter regions (six genes with σ D conditional binding and two genes with σ S conditional binding). Although in planktonic cells, six genes with condition-specific σ S binding showed elevated transcription levels comparing to electrogenic biofilm cells. As only a small number of differentially expressed genes are correlated with condition-specific σ factor regulation, it suggests that differential gene expression was not primarily regulated at the σ factor level in G. sulfurreducens . Additionally, binding profiles for σ S and σ N were analysed under early stationary phase and nitrogen-fixing conditions. The binding profiles of σ S and σ N were highly similar across these growth conditions as well ( Supplementary Data 1 ). For example, the binding profiles of σ S in exponentially grown cells were similar to early stationary phase (both planktonic cells), confirming that σ S is present and active under both exponential and stationary phases of growth in G. sulfurreducens ( Supplementary Fig. S4 ). σ S , different to its counterparts in other bacteria, regulated over 800 genes in the exponential phase where cells had sufficient nutrients and carbon supply. Almost 30% (254) of these genes were transcribed only from a σ S -dependent promoter under this condition ( Supplementary Data 4 ). This expanded role of σ S in exponential phase was further confirmed by comparing the transcriptomic profiles of a Δ rpoS strain and wild-type grown in exponential phase. Of the 254 genes transcribed solely from a σ S -dependent promoter, 96 genes were significantly downregulated by at least two-fold, while most others showed modest downregulation ( Supplementary Fig. S5a ; Supplementary Data 5 ). Genes that are directly related to nitrogen fixation were not transcribed when ammonium was used as nitrogen source, but were specifically activated under nitrogen limitation with binding of σ N in their promoter regions, indicating conditional binding and activity of σ N at these promoters. This conditional usage of σ N is likely due to the difference in the modulation of σ N activity. Unlike the other σ factors, the activity of σ N depends on the expression and binding of σ N -dependent transcription factors to σ N -targeted motifs. To further elucidate the functional state of the σ factor network, we assessed alternative usage of σ factors under the two divergent growth conditions (planktonic cells and electrogenic biofilm), and identified genes containing binding sites for multiple σ factors in the promoter region. Although the transcriptome changed by more than 10%, different σ factor usage at the same promoter region was not observed. Although the comparative analysis of the σ factor binding profiles suggests a near-static functional state of the σ factor network, functional enrichment of the different regulons indicated modularity in its operation. We integrated the genome-scale metabolic network [21] and transcriptomic differences between planktonic cells and electrogenic biofilm to provide an additional layer of context and insights into the effect of the σ factor network on the physiology of G. sulfurreducens . This analysis revealed that σ N and σ S primarily control energy metabolism during the shift from planktonic growth reducing fumarate to growth as an electrogenic biofilm, reiterating the trends observed from the functional enrichment analysis. Specifically, the gene encoding for DcuB, the terminal step in fumarate reduction, is regulated by σ N and its expression decreases by more than four-fold during the shift to electrogenic growth. Moreover, one of the outer membrane cytochromes essential for anode reduction (OmcZ) [26] is under σ N control and its expression level is upregulated during this particular shift. Additionally, σ N -controlled uptake hydrogenases that are not required for growth of G. sulfurreducens on the electrode were downregulated over eight-fold. As indicated in a previous study [27] , our analysis of binding profiles and transcriptomic data reaffirmed that σ S solely regulated the outer membrane cytochrome OmcB. This cytochrome is known to have an important role in extracellular electron transfer to the anode and was upregulated over 30-fold during this shift ( Fig. 4 ; Supplementary Data 3 ). On the other hand, σ D regulated biosynthetic processes that are critical during this particular growth shift. This is manifested in the two-fold increase in expression of a gene involved in iron–sulphur-cluster biosynthesis, recharge and transfer ( GSU2570 ) during growth as an electrogenic biofilm. These results indicate that the near-static functional state of the σ factor network mirrors the modularity of its operational state. 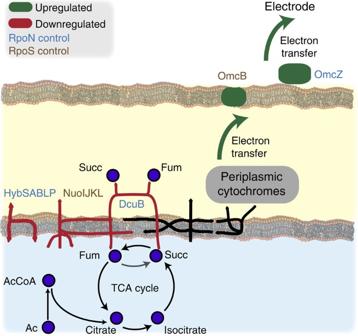Figure 4: Coordinated regulation of energy metabolism by alternative σ factors. Analysis of the differences in expression (two-fold change, FDR <0.5) and σ factor binding profiles between the two divergent growth conditions (planktonic cells and electrogenic biofilm) in the context of the genome-scale metabolic network. A snapshot of the key steps involved in the energy metabolism during this shift is shown. σNprimarily regulated energy metabolism during this shift by controlling the terminal steps in the respective respiratory processes (DcuB, and the outer membrane cytochrome OmcZ). σSregulated the NADH dehydrogenase (nuooperon) and the outer membrane cytochrome OmcB. The genes upregulated and downregulated in this shift are shown in green and red, respectively. OmcZ and NuoIJKL were also found to be co-regulated by σD. The alternative σ factors thus have a major role in the tight regulation of energy metabolism during this shift. It should be noted that this figure represents a snapshot of how the key genes involved in fumarate reduction and electrogenic biofilm growth are regulated by σ factors and not a mechanistic representation of the extracellular electron transfer pathway to the electrode. Figure 4: Coordinated regulation of energy metabolism by alternative σ factors. Analysis of the differences in expression (two-fold change, FDR <0.5) and σ factor binding profiles between the two divergent growth conditions (planktonic cells and electrogenic biofilm) in the context of the genome-scale metabolic network. A snapshot of the key steps involved in the energy metabolism during this shift is shown. σ N primarily regulated energy metabolism during this shift by controlling the terminal steps in the respective respiratory processes (DcuB, and the outer membrane cytochrome OmcZ). σ S regulated the NADH dehydrogenase ( nuo operon) and the outer membrane cytochrome OmcB. The genes upregulated and downregulated in this shift are shown in green and red, respectively. OmcZ and NuoIJKL were also found to be co-regulated by σ D . The alternative σ factors thus have a major role in the tight regulation of energy metabolism during this shift. It should be noted that this figure represents a snapshot of how the key genes involved in fumarate reduction and electrogenic biofilm growth are regulated by σ factors and not a mechanistic representation of the extracellular electron transfer pathway to the electrode. Full size image In eubacteria, σ factors have a critical role in transcriptional initiation by conferring promoter-binding specificity to the bacterial RNA polymerase. Understanding the complex network formed by the housekeeping and alternative σ factors and their regulons is foundational to elucidate mechanisms of transcriptional regulation and to realize the genotype–phenotype relationship. Here, we determined the topology, characterized the operational state and analysed its effect on the functional state of the network ( Fig. 5 ). This comprehensive network covers >80% of the genome and provides a framework to reconstruct the complete transcriptional regulatory network in this organism. 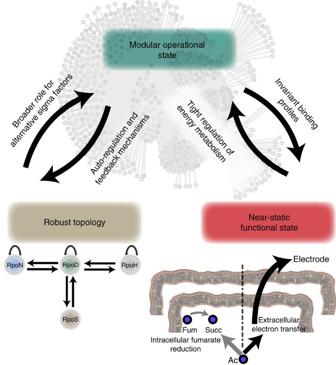Figure 5: Interplay between the multiple levels of σ factor network organization. The topology of the σ factor network inG. sulfurreducenssuggests a broader role for alternative σ factors. This resulted in a modular operational state with σNprimarily regulating genes involved in energy metabolism and maintaining redox homeostasis, while the housekeeping σDregulated biosynthetic processes. The σ factor network has a near-static functional state with invariant binding profiles between the two divergent growth conditions (planktonic cells and electrogenic biofilm). Analysis of the transcriptomic changes and σ factor binding profiles during this shift indicated that the necessitated tight regulation of energy metabolism during this shift is mirrored in the modularity of the operational state. This coordinated regulation in the operational state can further be attributed to the intertwined topology of the σ factor network where the major σ factors auto-regulate each other providing feedback mechanisms to fine-tune expression. Figure 5: Interplay between the multiple levels of σ factor network organization. The topology of the σ factor network in G. sulfurreducens suggests a broader role for alternative σ factors. This resulted in a modular operational state with σ N primarily regulating genes involved in energy metabolism and maintaining redox homeostasis, while the housekeeping σ D regulated biosynthetic processes. The σ factor network has a near-static functional state with invariant binding profiles between the two divergent growth conditions (planktonic cells and electrogenic biofilm). Analysis of the transcriptomic changes and σ factor binding profiles during this shift indicated that the necessitated tight regulation of energy metabolism during this shift is mirrored in the modularity of the operational state. This coordinated regulation in the operational state can further be attributed to the intertwined topology of the σ factor network where the major σ factors auto-regulate each other providing feedback mechanisms to fine-tune expression. Full size image Using the transcription unit architecture, we determined that the housekeeping σ D has over 2,000 genes in its regulon, and the other three alternative σ factors each regulate the expression of ~25% of the G. sulfurreducens genome. The experimentally determined transcription unit architecture and σ factor regulons further enabled us to elucidate the binding motifs of these four major σ factors. The binding motifs of the three σ 70 family σ factors (σ D , σ H and σ S ) closely resembled the classic σ factor binding motifs in bacteria, but show slight differences in individual base pairs within the motifs ( Supplementary Fig. S6 ). The motif of σ N is comparable to the known σ N motif described in other bacteria ( Supplementary Fig. S6 ). The reconstructed network further revealed that all of the alternative σ factors in G. sulfurreducens regulate the housekeeping σ D , thereby forming a highly intertwined network. Another unexpected feature of this σ factor network is the auto-regulation of its σ factors. Both σ N and σ H auto-regulate their own expression, which is not the case in E. coli , but known in other bacteria, such as in Rhizobium leguminosarum (σ N ) [28] and Caulobacter crescentus (σ H ) [29] . This feature could influence the operation of the σ factor network in G. sulfurreducens by providing a direct feedback mechanism to fine-tune its σ factor transcription levels. In addition, the topology of the σ factor network suggests a greater role for alternative σ factors than what has been reported for E. coli or B. subtilis [18] ( Supplementary Note 1 ). This topological feature resulted in a modular operational state with σ N primarily regulating genes involved in energy metabolism and maintaining redox homeostasis, while the housekeeping σ D regulated biosynthetic processes. Contrary to its typical role of controlling stress response [30] , the regulon of σ S in G. sulfurreducens was enriched for regulating energy metabolism. Consistent with this functional difference, the activity and protein levels of σ S were almost unchanged between exponential and stationary growth phase ( Supplementary Fig. S4 ), a feature typically exhibited by housekeeping σ factors. However, the size of RpoS (~40 kDa) [31] and its binding motif are typical of bacterial σ S ( Supplementary Figs S4 and S6 ). Taken together, the lack of auto-regulation and a capability to regulate other σ factors further preclude classification of this σ S homologue as an alternative housekeeping σ factor. It could be speculated that another σ factor, particularly σ E , controls the main stress response in G. sulfurreducens . However, induction of σ E was neither observed under stationary phase growth nor during heat or cold shock, suggesting a limited role of σ E under these conditions. Furthermore, we compared the transcriptome of cells grown in exponential and early stationary phase. Among the 254 genes that only have σ S binding sites identified in their promoter regions, most of them exhibited modest upregulation in early stationary phase compared with exponential phase ( Supplementary Fig. S7 ; Supplementary Data 5 ). The most upregulated genes in early stationary phase are iron–sulphur containing proteins and genes related to ferrous iron transport, (for example, the fur-feoB-ideR operon). However, these genes were not under σ S regulation, but rather transcribed from σ D and/or σ N controlled promoters. This leads us to postulate that there is no designated σ factor in G. sulfurreducens that is predominantly active under stationary phase growth. Systems-level analysis of transcriptomic changes and comparative binding profiles between the most divergent growth conditions attributed this difference in the functional state to topological and operational properties of the σ factor network. In G. sulfurreducens, σ D regulates biosynthetic processes and other housekeeping functions, while σ N is the primary σ factor that regulates energy metabolism to maintain redox homeostasis. The two divergent growth conditions evaluated here represent very different modes of respiration, with electrogenic biofilm growth requiring extracellular electron transfer as opposed to intracellular fumarate reduction during planktonic growth. Both these growth modes necessitate a tight regulation of energy metabolism and maintenance of redox homeostasis, unlike the shift from respiration to fermentation in E. coli . Thus, the modular operational state is fundamental to the tight regulation of energy metabolism manifested in this near-static functional state of the σ factor network. This is likely a consequence of the potential feedback mechanisms revealed by the intertwined topology of the network ( Fig. 5 ). Genetic alteration of the network might provide insights into the mechanisms modulating the σ factor network of G. sulfurreducens ( Supplementary Note 1 ). Further comparison of the interaction between σ factors and major transcriptional regulators in G. sulfurreducens and E. coli ( Supplementary Fig. S8 ), revealed that the majority of transcriptional regulators in G. sulfurreducens (51%) are under shared regulation by multiple σ factors (compared with 23% in E. coli ). Moreover, 44% of the transcription factors in E. coli are solely regulated by σ D (24% in G. sulfurreducens ), with alternative σ factors having a peripheral role in regulation of transcription factors. Thus, it is possible that in a tightly controlled near-static σ factor network, like that of G. sulfurreducens , the dynamic response of the organism to environmental stimuli occurs predominantly at the level of the transcriptional regulatory network ( Fig. 5 ). In summary, we have experimentally reconstructed a comprehensive σ factor regulatory network in G. sulfurreducens . The topology of this network is different from what has been described so far for other bacteria. In addition to the topology, the detailed characterization of the operational state highlighted critical functional differences between the σ factor network of a specialist like G. sulfurreducens and a generalist like E. coli . Analysing the σ factor regulatory network in the light of a comprehensive transcription unit architecture provides a framework to map binding activities of transcription factors as well as regulatory events of small signal molecules and will further our understanding of principles underlying transcription regulatory networks in bacteria. Bacterial strains and growth conditions Wild-type G. sulfurreducens (ATCC 51573) and a Δ rpoS strain [31] were grown under strictly anoxic conditions at 30 °C with acetate as electron donor and fumarate or ferric citrate as electron acceptor as previously described [32] . Cell growth was monitored by measuring OD 600 . When ferric citrate was used as electron acceptor, cell growth was determined by measuring Fe(II) concentration in the medium and correlated to protein content. For growth in the absence of fixed inorganic nitrogen, ammonium chloride was omitted from the medium and N 2 served as the only nitrogen source. Cells in microbial fuel cells were grown as described previously [33] . For heat shock condition, cells were grown with acetate as electron acceptor and fumarate as electron donor. Cells (100 ml) were grown at 30 °C in 160 ml serum bottles until mid-exponential phase and then incubated in a 42-°C water bath for 15 min before processing. ChIP-chip and ChIP-seq ChIP-chip for RpoD was performed as described previously [9] . ChIP-chip for RpoH, RpoN and RpoS was carried out identical as described for RpoD but with polyclonal antibodies generated using rabbits as host animals. Genome-wide σ factor binding sites were determined for cells grown under various conditions. Before microarray hybridization, real-time quantitative PCR targeting previously known binding regions were carried out to verify enrichment of IP DNA fragments. qPCR and amplification of DNA was performed as previously described [8] . Microarray hybridization, wash and scan were performed in accordance with manufacturer’s instruction (Roche Nimblegen). ChIP-seq was performed with NEBNext ChIP-Seq Library Prep Master Mix Set for Illumina (NEB) with indexed adaptors (Illumina). Sequencing was performed with a GAII sequencer (Illumina) by the UCSD Biogem facility. Sequence data were then aligned onto the G. sulfurreducens PCA genome (NC_002939) using Mosaik Aligner ( http://bioinformatics.bc.edu/marthlab/Mosaik ) with two mismatch allowed in each read. Transcriptome profiling by RNA-seq Wild-type and Δ rpoS cells of G. sulfurreducens were harvested from mid-exponential (OD 600 =0.25) and early stationary phase with acetate as electron donor and fumarate as electron acceptor. Total RNA was isolated using TRIzol reagent (Invitrogen). Residual DNA was removed with a 30-min DNAse I digestion at 37 °C (Qiagen) followed by purification with RNeasy Mini kit (Qiagen). A total of 2.5 μg of total RNA was treated with the Gram-negative RiboZero kit (Epicentre). Paired end, strand-specific RNA sequencing was performed using a variation of the dUTP method [34] , [35] with the following changes: 100 ng of rRNA subtracted RNA was fragmented with RNA fragmentation reagents (Ambion) for 2.5 min at 70 °C. First-strand synthesis was primed using random hexamers (Invitrogen). Downstream library construction was performed as previously described [36] . Indexed PCR primers were used for library amplification. Libraries were then quantified using a 2100 Bioanalyzer (Agilent) and sequenced on a MiSeq (Illumina). The obtained RNA-seq reads were aligned to the genome sequence of G. sulfurreducens (RefSeq NC_002939) using the short-read aligner Bowtie [37] with two mismatches allowed per read alignment. To estimate transcript abundances, FPKM values were calculated by using Cufflinks ( http://cufflinks.cbcb.umd.edu/ ) [38] with appropriate parameters set for the strand-specific library type and upper-quartile normalization. Pair-wise differential expression analysis was carried out using Cuffdiff, with upper-quartile normalization and appropriate parameters set for strand-specific library type. A fold change of greater than two-fold and false-discovery rate cutoff of 0.05 was used to determine significant differential expression between two different conditions. Identification of σ factor binding regions Binding regions of σ factors were determined with both NimbleScan software as described before [9] and MA2C [17] . Band width equals to 250, and FDR equals to 0.05 was used in MA2C. Negative control regions were randomly selected from known non-binding regions. Binding regions called in both software packages were manually curated and then used in downstream analysis. Identification of σ factor binding motifs For each σ factor, binding regions that were upstream a transcription start site (TSS) and not overlapping with binding sites of other σ factors were used as input. The motif was first determined by MEME [39] , then refined by Bioprospector [40] . Bacterial promoters can be grouped into two different families. The σ D σ factor family includes the housekeeping σ D as well as most of the alternative σ factors, such as σ H and σ S . The binding motifs for this σ factor family are generally composed of two consensus sequences centred at around −10 and −35 from the TSS [1] . The second family that contains σ N , contains −24/−12 type promoters [1] . Promoters from both families are composed of multiple conserved elements, which are separated by variable length spacers, making them hard to predict computationally. Our experimentally identifying σ factor binding regions in G. sulfurreducens consequently allowed elucidating the σ factor binding motifs unambiguously. For each σ factor, binding regions that were not shared with other σ factors and additionally contained an experimentally determined TSS were considered. MEME [39] was used for initial motif scan to determine the right parameters for BioProspector. BioProspector [40] were then used to identify potential two-part motifs. The results showed that all σ factors belonging to the σ D familiy (σ D , σ H , σ S ) contained a −35 element (TTGAC) that closely resemble the classic bacterial σ D −35 element (TTGACA), with a less conserved −10 motif (TANNNT) ( Supplementary Fig. S2 ). The binding motif determined for σ S had the least conserved −35 element within this family, but exhibited a relatively strong −10 and an extended −10 element (G at −14). σ H has both strong −10 and −35 element but may due to limited number of σ H only promoters identified. It is known that many cis promoter elements can contribute to promoter selectivity of different σ factors. For example, σ S promoters in E. coli contain a hallmark C base at position −13 to make the promoter preferable to σ S because of different charged amino acid located at the beginning of the domain 3 alpha helix [41] . The subtle differences in the σ factor binding motifs in G. sulfurreducens are very likely to contribute to the σ factor selectivity at different σ D family promoters in vivo . The determined binding motif for σ N family promoters resembled the classic −24/−12 type motif found in other bacteria. It is known that the activities of σ N promoters are modulated by an enhancer-dependent mechanism, and the selective expression of σ N promoters under different conditions in G. sulfurreducens could depend on the activity of the 30 predicted σ N -dependent enhancers encoded in the G. sulfurreducens genome [42] . Western blot Cells were harvested, pelleted via centrifugation and if not processed immediately, frozen at −80 °C until further use. Samples were resuspended in LDS sample buffer (Invitrogen) containing 10 × reducing agent (Invitrogen) based on optical density in order to normalize protein content. Each sample was lysed at 95 °C for 5 min and subjected to electrophoresis on a 10% polyacrylamide gel (Invitrogen). Resolved proteins were electrotransferred to a Hybond-ECL membrane (Amersham Biosciences). Nonspecific binding was prevented by incubating the ECL membrane in nonfat dried milk overnight. The ECL western detection kit, G. sulfurreducens RpoS polyclonal antibody and horseradish-peroxidase-conjugated donkey anti-rabbit immunoglobulin G (Amersham Biosciences) were used to detect the presence of RpoS. Functional enrichment analysis of the regulons The functional categories for the G. sulfurreducens genes were obtained from the subsystems assigned in the SEED database [20] . To determine if the regulons of each σ factor were significantly enriched for any particular functional category, a hypergeometric test was performed using the hygecdf function in MATLAB. A P -value cutoff of 0.05 was used to determine significance. In silico gene essentiality simulations Genes in the genome-scale metabolic model of G. sulfurreducens were individually knocked-out and in silico growth simulations were performed. This was achieved using the ‘singleGeneDeletion’ function of the COBRA toolbox [43] . Accession codes: All data have been deposited in the Gene Expression Omnibus database under the accession codes GSE22503 , GSE17837 , GSE22497 , GSE17834 and GSE37778 . How to cite this article: Qiu, Y. et al . Characterizing the interplay between multiple levels of organization within bacterial σ factor regulatory networks. Nat. Commun. 4:1755 doi: 10.1038/ncomms2743 (2013).